HIV-1 capsids bind and exploit the kinesin-1 adaptor FEZ1 for inward movement to the nucleus Intracellular transport of cargos, including many viruses, involves directed movement on microtubules mediated by motor proteins. Although a number of viruses bind motors of opposing directionality, how they associate with and control these motors to accomplish directed movement remains poorly understood. Here we show that human immunodeficiency virus type 1 (HIV-1) associates with the kinesin-1 adaptor protein, Fasiculation and Elongation Factor zeta 1 (FEZ1). RNAi-mediated FEZ1 depletion blocks early infection, with virus particles exhibiting bi-directional motility but no net movement to the nucleus. Furthermore, both dynein and kinesin-1 motors are required for HIV-1 trafficking to the nucleus. Finally, the ability of exogenously expressed FEZ1 to promote early HIV-1 infection requires binding to kinesin-1. Our findings demonstrate that opposing motors both contribute to early HIV-1 movement and identify the kinesin-1 adaptor, FEZ1 as a capsid-associated host regulator of this process usurped by HIV-1 to accomplish net inward movement towards the nucleus. Free diffusion is severely impeded inside the dense cell cytosol and, as such, directed long-range movement of macromolecules is mediated by microtubules (MTs). MTs consist of α/β-tubulin subunits arranged into polarized filaments whose minus-ends are usually anchored at the centrosome, the primary microtubule-organizing centre in many cells types, whereas their plus-ends radiate towards the cell periphery. Specific motor complexes bind cargos and direct their movement on MTs. Generally, minus-end directed (retrograde) movement is driven by dynein while plus-end directed (anterograde) motion is driven by kinesins [1] . Motor-mediated transport of macromolecules and organelles plays important roles in a wide range of processes including cell polarization and migration, as well as infection by a variety of pathogens including human immunodeficiency virus type 1 (HIV-1) [2] . HIV-1 is a retrovirus that causes AIDS. The events occurring immediately after HIV-1 entry into the host cell are complex and one of the most poorly understood aspects of the viral life cycle. It is known that after core particles enter the cytosol the viral single-stranded RNA genome is reverse transcribed into double-stranded DNA that then enters the nucleus through nuclear pore proteins and, ultimately, integrates into the host chromosome [3] . Virus uncoating and reverse transcription is thought to occur either while the virus is being transported along MTs or upon reaching the nucleus [4] , [5] , [6] . When expressed in yeast HIV-1 integrase also traffics in a MT- and dynein-dependent manner [7] . However, whether this is due to a direct interaction of HIV-1 core proteins with dynein components or there is an indirect ‘piggy back’ association of incoming cores is unclear. Our previous work exploring the resistance of a chemically mutagenized cell line to retroviral infection identified the causal gene as fasciculation and elongation protein zeta-1 ( FEZ1 ) [8] . FEZ1 did not affect viral entry into the cell but specifically inhibited the accumulation of circularized viral DNA, an indicator of retroviral DNA entry into the nucleus [8] . In addition, we have shown that FEZ1 protein is expressed at very high levels in neurons and this contributes to their natural resistance to HIV-1 (ref. 9 ). However, the underlying mechanism of how FEZ1 affects the delivery of retroviral DNA to the nucleus and its potential role in infection of other cell types remains unknown. Here, we show that FEZ1 functions as a positive factor for HIV-1 infection of a number of non-neuronal cell types including natural target cell types for HIV-1. Our findings suggest that FEZ1 does not affect specific HIV-1 nuclear entry pathways but, instead, HIV-1 capsids bind FEZ1, a kinesin-1 adaptor protein, to regulate viral movement towards the nucleus. We show that early HIV-1 infection not only requires the inward motor, dynein, but also depends on the outward motor, kinesin-1. Furthermore, exogenous FEZ1 expression promotes early HIV-1 infection while a mutant of FEZ1 that does not bind kinesin-1 fails to do so. Our findings suggest that opposing motors contribute to bi-directional HIV-1 movement, and that incoming viral particles usurp the kinesin-adaptor function of the host protein, FEZ1, to regulate this process and accomplish net retrograde movement to the nucleus. FEZ1 promotes HIV-1 infection in non-neuronal cells Although naturally high FEZ1 levels contribute to neuronal resistance to HIV-1 infection [8] , [9] , the potential contribution of FEZ1 to infection in other cell types remains unknown. To begin exploring this, endogenous FEZ1 levels were measured in different human cell types by western blotting (WB). In line with our previous work, FEZ1 was naturally expressed at high levels in the neuroblastoma line, SH-SY5Y, compared with either the human microglia line, CHME3 or primary normal human dermal fibroblasts (NHDFs; Fig. 1a ). FEZ1 levels in a variety of T-cell and monocyte lines were also found to be either comparable with or lower than those in NHDFs ( Supplementary Fig. 1 ), demonstrating that FEZ1 expression in various natural target cell types (microglia, T cells and monocytes) and NHDFs is notably lower than in neuronal cells. To test if endogenous FEZ1 levels in non-neuronal cells could influence their susceptibility to infection, FEZ1 was depleted in NHDFs, microglia (CHME3) or macrophages (differentiated Thp-1) using RNA interference. Small interfering RNA (siRNA)-treated cells were then infected with HIV-1 carrying a luciferase reporter gene and pseudotyped with vesicular stomatitis virus G (VSV-G) envelope glycoprotein, widely used to improve HIV-1 infectivity and which mediates endocytic fusion, one of the entry pathways used by HIV-1 (refs 10 , 11 ). Measurements of luciferase activity revealed that compared with control siRNA-treated cultures, FEZ1 depletion using either of two independent siRNAs potently reduced HIV-1 infection in all three cell types ( Fig. 1b,d,f , respectively). Furthermore, WB analysis showed that effects on infection correlated with the levels of FEZ1 depletion achieved with each siRNA ( Fig. 1c,e,g ). Although FEZ1 siRNAs did not affect cell morphology or induce apoptosis ( Supplementary Fig. 2a and 2b , respectively), to further rule out potential off-target effects, the ability of exogenously expressed siRNA-resistant flag-tagged FEZ1 to rescue infection was tested. In control Flag-expressing NHDFs, FEZ1 siRNAs reduced FEZ1 levels and suppressed HIV-1 infection ( Fig. 1h,i ). By contrast, FEZ1 levels were maintained in FEZ1-Flag-expressing NHDFs in the presence of FEZ1 siRNAs and infectivity was restored ( Fig. 1h,i ). Again, the levels of viral infection correlated directly with the levels of FEZ1 expression. 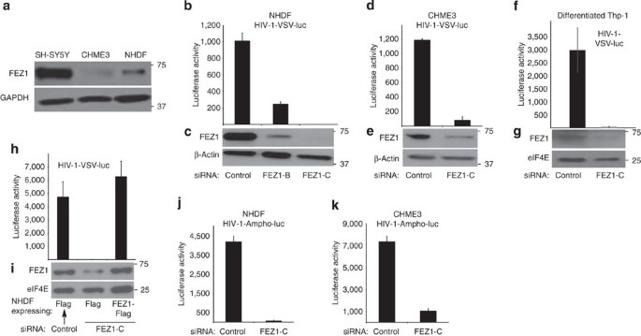Figure 1: FEZ1 is a positive regulator of HIV-1 infection in non-neuronal human cells. (a) Endogenous levels of FEZ1 in neuroblastoma cells (Sh-SY5Y), microglia (CHME3) or primary normal human dermal fibroblasts (NHDF). Equal cell numbers were lysed and analysed by WB using anti-FEZ1 antibody. Equal loading was confirmed using anti-GAPDH antibody. (b–i) FEZ1 is required for early HIV-1 infection regardless of the route of viral entry. NHDF (b,c), CHME3 (d,e) or Thp-1 differentiated into macrophages (f,g) were transfected with control siRNA (control) or independent FEZ1 siRNAs (FEZ1-B or FEZ1-C). Forty-eight hours post transfection cells were infected with HIV-1-VSV-luc followed by measurements of luciferase activity to determine levels of infection in NHDF (b), CHME3 (d) or differentiated Thp-1 (f) cells. (c,e,g) WB analysis showing the extent of FEZ1 depletion in samples fromb,dandf, respectively. β-Actin or eIF4E were used as loading controls. (h,i) Rescue of RNA interference-mediated FEZ1 depletion restores HIV-1 infection. (h) Pools of NHDF cells expressing either Flag control or FEZ1-Flag were treated with either control or FEZ1-C siRNAs followed by HIV-1-VSV-luc infection and measurements of infectivity as inb–d. (i) WB analysis showing the levels of FEZ1 in samples fromh. eIF4E was used as a loading control. (j,k) NHDF or CHME3 cells were transfected with control or FEZ1-C siRNAs followed by infection with HIV-1-Ampho-luc 48 h post-transfection. Luciferase assays were used to determine levels of infection in NHDF (j) or CHME3 (k). Results are representative of three or more independent experiments, and error bars represent standard deviation. Molecular weight markers (in kDa) are shown to the right of WBs. Figure 1: FEZ1 is a positive regulator of HIV-1 infection in non-neuronal human cells. ( a ) Endogenous levels of FEZ1 in neuroblastoma cells (Sh-SY5Y), microglia (CHME3) or primary normal human dermal fibroblasts (NHDF). Equal cell numbers were lysed and analysed by WB using anti-FEZ1 antibody. Equal loading was confirmed using anti-GAPDH antibody. ( b – i ) FEZ1 is required for early HIV-1 infection regardless of the route of viral entry. NHDF ( b , c ), CHME3 ( d , e ) or Thp-1 differentiated into macrophages ( f , g ) were transfected with control siRNA (control) or independent FEZ1 siRNAs (FEZ1-B or FEZ1-C). Forty-eight hours post transfection cells were infected with HIV-1-VSV-luc followed by measurements of luciferase activity to determine levels of infection in NHDF ( b ), CHME3 ( d ) or differentiated Thp-1 ( f ) cells. ( c , e , g ) WB analysis showing the extent of FEZ1 depletion in samples from b , d and f , respectively. β-Actin or eIF4E were used as loading controls. ( h , i ) Rescue of RNA interference-mediated FEZ1 depletion restores HIV-1 infection. ( h ) Pools of NHDF cells expressing either Flag control or FEZ1-Flag were treated with either control or FEZ1-C siRNAs followed by HIV-1-VSV-luc infection and measurements of infectivity as in b – d . ( i ) WB analysis showing the levels of FEZ1 in samples from h . eIF4E was used as a loading control. ( j , k ) NHDF or CHME3 cells were transfected with control or FEZ1-C siRNAs followed by infection with HIV-1-Ampho-luc 48 h post-transfection. Luciferase assays were used to determine levels of infection in NHDF ( j ) or CHME3 ( k ). Results are representative of three or more independent experiments, and error bars represent standard deviation. Molecular weight markers (in kDa) are shown to the right of WBs. Full size image HIV-1 can also enter cells by membrane fusion [11] , which can be mimicked by pseudotyping HIV-1 with murine leukemia virus (MuLV) amphotropic envelope [12] , [13] . Similar to HIV-1-VSV-luc, FEZ1 depletion also blocked infection by HIV-1-Ampho-luc in both NHDF and CHME3 cells ( Fig. 1j,k , respectively). This demonstrated that FEZ1 regulates HIV-1 infection regardless of the route of viral entry, similar to our previous findings that FEZ1 regulates post-entry stages of HIV-1 infection [8] , [9] . These findings also demonstrated that FEZ1 positively regulates HIV-1 infection in non-neuronal primary human cells and natural target cells such as microglia and macrophages. Furthermore, although increasing expression of exogenous FEZ1-Flag increased infectivity in NHDFs, this effect began to decline in cells expressing very high levels of FEZ1 ( Supplementary Fig. 3a and b ). This suggests that FEZ1’s antiviral activity previously observed in neurons is likely due to excessively high levels in these cells [9] , as discussed later. FEZ1 regulates the movement of incoming HIV-1 Although our previous findings suggested that FEZ1 affects infection at or before nuclear entry [8] , [9] , the underlying mechanism remains unknown. Given that FEZ1 acts as a cargo adaptor and affects early stages of infection, we tested whether FEZ1 might bind in vitro assembled HIV-1 capsid-nucleocapsid (CA–NC) complexes [14] , [15] . Extracts from cells expressing C-terminally Flag-tagged FEZ1 were mixed with assembled capsids that were then sedimented by centrifugation. As shown in Fig. 2a , FEZ1-Flag was found to associate with HIV-1 CA–NC complexes as was a C-terminally Flag-tagged cytoplasmically localized version of the cleavage and polyadenylation specificity factor subunit 6 (NES-CPSF6-Flag) protein, also known to bind HIV-1 particles [15] , [16] . By contrast, Flag-tagged SAM domain and HD domain-containing protein (SAMHD1) [17] did not bind, demonstrating the specificity of the FEZ1 association. FEZ1 was also independently found to co-immunoprecipitate (Co-IP) with HIV-1 Gag, the viral structural polyprotein containing matrix, capsid and nucleocapsid, below. These findings suggested that FEZ1 could associate with incoming HIV-1 particles and potentially affect a number of early steps in the viral lifecycle, such as capsid-mediated nuclear import [3] . HIV-1 exploits nuclear entry pathways involving TNPO3 and/or NUP358 (ref. 18 ). Recently, two capsid mutants, termed N74D and P90A, were shown to mediate entry into the nucleus independently of NUP358 and/or transportin pathways [19] . As such, if FEZ1 specifically affected HIV-1 nuclear entry pathways then these two capsid mutants should be able to bypass FEZ1 activity. To test this, NHDFs treated with control or FEZ1-targeting siRNAs were infected using pseudotyped HIV-1 composed of wild type (WT; p8.91), N74D or P90A capsids. WT or capsid mutant viruses were titred by ELISA analysis of p24 capsid protein levels in stock preparations of each virus and dilutions were used to ensure equal amounts of virions were used for infections. Again, FEZ1 depletion in primary fibroblasts, confirmed by WB ( Fig. 2b ), potently blocked infection with HIV-1 regardless of whether the virus had WT ( Fig. 2c ), N74D ( Fig. 2d ) or P90A ( Fig. 2e ) capsid. Although this does not rule out the possibility that FEZ1 might regulate multiple independent nuclear entry pathways to influence infection by each of these viruses, these findings demonstrated that FEZ1’s effects on HIV-1 infection could not be bypassed by changing the route of nuclear entry and suggested that FEZ1 was not directly involved in nuclear entry pathways specifically used by HIV-1. 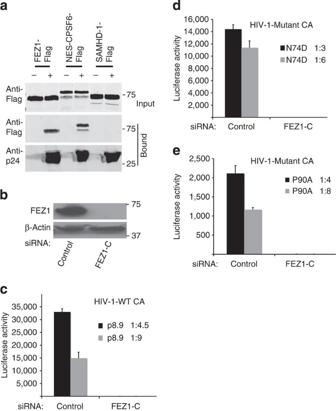Figure 2: FEZ1 bindsin vitroassembled HIV-1 CA–NC complexes and affects infection. (a) Binding of FEZ1 toin vitroassembled HIV-1 CA–NC complexes. 293T cells were transfected with plasmids expressing C-terminally flag-tagged FEZ1 (FEZ1-Flag), C-terminally flag-tagged CPSF6 (NES-CPSF6-Flag) or C-terminally flag-tagged SAMHD1 (SAMHD1-Flag). Cells were lysed 36 h post transfection and the lysates were incubated at room temperature for 1 h within vitroassembled HIV-1 CA–NC complexes. Samples were taken either before (input) or after sedimentation through a 70% sucrose cushion (bound) and analysed by WB using anti-Flag and anti-p24 antibodies. (b–e) Effects of FEZ1 depletion on HIV-1 carrying WT or mutant caspids. NHDF cells were transfected with control siRNA or FEZ1 siRNA (FEZ1-C). Forty-eight hours post transfection, cells were (b) lysed and analysed by WB using antibodies to FEZ1 or β-actin (loading control) or (c–e) siRNA-transfected cells were infected with different dilutions of HIV-1-VSV-luc carrying a WT (p8.91) (c), N74D (d) and P90A (e) capsid. Forty-eight hours post infection, luciferase activity was used to determine levels of infection. Results are representative of three or more independent experiments, and error bars represent standard deviation. Molecular weight markers (in kDa) are shown to the right of WBs. Figure 2: FEZ1 binds in vitro assembled HIV-1 CA–NC complexes and affects infection. ( a ) Binding of FEZ1 to in vitro assembled HIV-1 CA–NC complexes. 293T cells were transfected with plasmids expressing C-terminally flag-tagged FEZ1 (FEZ1-Flag), C-terminally flag-tagged CPSF6 (NES-CPSF6-Flag) or C-terminally flag-tagged SAMHD1 (SAMHD1-Flag). Cells were lysed 36 h post transfection and the lysates were incubated at room temperature for 1 h with in vitro assembled HIV-1 CA–NC complexes. Samples were taken either before (input) or after sedimentation through a 70% sucrose cushion (bound) and analysed by WB using anti-Flag and anti-p24 antibodies. ( b – e ) Effects of FEZ1 depletion on HIV-1 carrying WT or mutant caspids. NHDF cells were transfected with control siRNA or FEZ1 siRNA (FEZ1-C). Forty-eight hours post transfection, cells were ( b ) lysed and analysed by WB using antibodies to FEZ1 or β-actin (loading control) or ( c – e ) siRNA-transfected cells were infected with different dilutions of HIV-1-VSV-luc carrying a WT (p8.91) ( c ), N74D ( d ) and P90A ( e ) capsid. Forty-eight hours post infection, luciferase activity was used to determine levels of infection. Results are representative of three or more independent experiments, and error bars represent standard deviation. Molecular weight markers (in kDa) are shown to the right of WBs. Full size image The association of FEZ1 with HIV-1 might also affect the movement of incoming virus to the nucleus, rather than playing a direct role in the nuclear entry process. Indeed, FEZ1 is known to act as a kinesin-1 adaptor protein [20] . To test this, the potential effects of FEZ1 depletion on the movement of HIV-1 particles carrying GFP-tagged Vpr [4] were examined. Live imaging of virus in cells treated with either control or FEZ1 siRNAs revealed that in both cases viral particles exhibited long-range bi-directional motility ( Supplementary Movies 1–3 , respectively). Similar bi-directional movement was observed in microglia ( Supplementary Movie 4 ), and has been reported in other cell types [4] , [5] , demonstrating that this was not unique to NHDFs. Movies and still images generated from these movies suggested that the majority of particles observed in control siRNA-treated NHDFs gradually moved towards the nucleus ( Supplementary Movie 1 and Fig. 3a , upper panels). However, viral particles in FEZ1-depleted cells frequently appeared to make progress towards the nucleus before suddenly making long runs back towards the cell periphery ( Supplementary Movies 2 and 3 and Fig. 3a , lower panels). To confirm this, cells were treated and infected as above but imaged at a higher frame rate of 2 frames per second over a 150-s period. Measuring distances travelled by viral particles in either retrograde or anterograde directions revealed that in control siRNA-treated cells particles on average travelled longer retrograde than anterograde distances resulting in a net ~1 μm movement towards the nucleus in this time ( Fig. 3b ). By contrast, in FEZ1-depleted cells, viral particles on average travelled longer anterograde distances, resulting in net ~1.5 μm movement towards the cell periphery ( Fig. 3b ). In line with these observations, measuring the distance of viral particles from the nucleus revealed that although the number of viral particles reaching within 2 μm of the nucleus increased over time in control siRNA-treated cells (particle numbers gradually decline from their peak, likely due to uncoating, nuclear entry and/or photobleaching at later stages), the majority of viral particles failed to reach within 2 μm of the nucleus in FEZ1-depleted cells ( Fig. 3c ). Finally, to distinguish viral particles that had fused into the cytoplasm from those that might have been non-productively endocytosed, control or FEZ1 siRNA-treated cells were infected with VSV-G-pseudotyped double-labelled virus composed of Vpr-GFP (labelling the viral core) and S15-Tomato (labelling the viral membrane) [21] . Unfused viral particles appear yellow, whereas fused particles shed the S15-Tomato-labelled viral membrane and appear green. As shown in Fig. 3d,e , FEZ1 depletion did not affect the number of green particles in the cell but decreased the number of fused (green) viral particles within 2 μm of the nucleus compared with controls. Confirming that these green particles represented fused virus, their number as a percentage of total viral particles in the cell was significantly reduced by treatment of cells with the fusion inhibitor, Bafilomycin ( Fig. 3f ), similar to previous reports [22] . These data collectively demonstrated that FEZ1 associated with in vitro assembled HIV-1 CA–NC complexes and was required for efficient movement of HIV-1 across the cytoplasm to the nucleus. 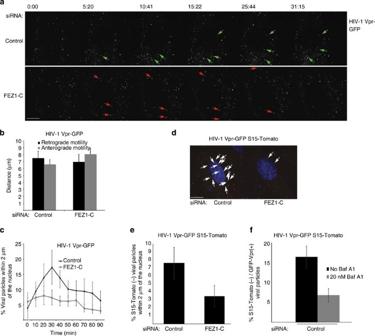Figure 3: Depletion of FEZ1 inhibits HIV-1 trafficking to the nucleus. NHDFs were treated with control or FEZ1-C siRNAs. Forty-eight hours post transfection, cells were infected with HIV-1-VSV-GFP-Vpr followed by live imaging using a spinning-disc confocal microscope. (a) Still images from movies (Supplementary Movies 1 and 2) taken at the indicated times are shown. Green arrows highlight viral particles entering and traversing the cytoplasm in control siRNA-treated cells. Red arrows highlight representative examples of particles that approach the nucleus but then move long distances back out to the cell periphery in FEZ1-depleted cells. (b) Quantification of the average distance (μm per 2.5 min) travelled by viral particles towards the nucleus (Retrograde motility) or away from the nucleus (Antrograde motility).n≥5 cells and an average of 7–30 viral particles per cell. (c) Quantification of the percentage of virions within 2 μm of the nucleus in infected siRNA-treated cells at the indicated time points.n≥20 cells and an average of 80–99 viral particles per cell. (d–f) Depletion of FEZ1 affects HIV-1 particles that have productively fused into the cytoplasm. (d) NHDF cells were treated with control or FEZ1-C siRNAs. Forty-eight hours after transfection, cells were infected with HIV-1-VSV containing GFP-Vpr and S15-Tomato. One hour post infection, cells were fixed in formaldehyde and GFP and Tomato signals were acquired using a spinning-disc confocal microscope. Arrows highlight fused (green, S15-negative) particles proximal to the nucleus in each sample. Representative confocal planes are shown. (e) Quantification of the % fused (green, S15-negative) viral particles within 2 μm of the nucleus in samples as described and processed ind.n≥29 cells and an average of 53–55 viral particles per cell. (f) Control siRNA-treated NHDF cells were treated with Bafilomycin A1 for 2 h during spinoculation followed by infection with HIV-1-VSV containing GFP-Vpr and S15-Tomato. One hour post infection, cells were fixed and the total number of fused (green, S15-negative) viral particles were quantified and presented as a % of the total number of viral particles.n≥29 cells and an average of 55–80 viral particles per cell. Error bars represent standard deviation. Scale bars represent 10 μm. Figure 3: Depletion of FEZ1 inhibits HIV-1 trafficking to the nucleus. NHDFs were treated with control or FEZ1-C siRNAs. Forty-eight hours post transfection, cells were infected with HIV-1-VSV-GFP-Vpr followed by live imaging using a spinning-disc confocal microscope. ( a ) Still images from movies ( Supplementary Movies 1 and 2 ) taken at the indicated times are shown. Green arrows highlight viral particles entering and traversing the cytoplasm in control siRNA-treated cells. Red arrows highlight representative examples of particles that approach the nucleus but then move long distances back out to the cell periphery in FEZ1-depleted cells. ( b ) Quantification of the average distance (μm per 2.5 min) travelled by viral particles towards the nucleus (Retrograde motility) or away from the nucleus (Antrograde motility). n ≥5 cells and an average of 7–30 viral particles per cell. ( c ) Quantification of the percentage of virions within 2 μm of the nucleus in infected siRNA-treated cells at the indicated time points. n ≥20 cells and an average of 80–99 viral particles per cell. ( d – f ) Depletion of FEZ1 affects HIV-1 particles that have productively fused into the cytoplasm. ( d ) NHDF cells were treated with control or FEZ1-C siRNAs. Forty-eight hours after transfection, cells were infected with HIV-1-VSV containing GFP-Vpr and S15-Tomato. One hour post infection, cells were fixed in formaldehyde and GFP and Tomato signals were acquired using a spinning-disc confocal microscope. Arrows highlight fused (green, S15-negative) particles proximal to the nucleus in each sample. Representative confocal planes are shown. ( e ) Quantification of the % fused (green, S15-negative) viral particles within 2 μm of the nucleus in samples as described and processed in d . n ≥29 cells and an average of 53–55 viral particles per cell. ( f ) Control siRNA-treated NHDF cells were treated with Bafilomycin A1 for 2 h during spinoculation followed by infection with HIV-1-VSV containing GFP-Vpr and S15-Tomato. One hour post infection, cells were fixed and the total number of fused (green, S15-negative) viral particles were quantified and presented as a % of the total number of viral particles. n ≥29 cells and an average of 55–80 viral particles per cell. Error bars represent standard deviation. Scale bars represent 10 μm. Full size image Kinesin-1 is required for early HIV-1 infection To further explore how a kinesin-1 adaptor protein might regulate net inward movement of HIV-1, we examined whether kinesin-1 itself contributed to early infection. To do this, siRNAs were used to deplete different human cell types of either of two different isoforms of kinesin-1 heavy chain, Kif5A or Kif5B, followed by infection of these cells with HIV-1-VSV-luc reporter. Knockdown of either Kif5A or Kif5B inhibited infection in both primary fibroblasts (NHDFs; Fig. 4a ) and human microglia (CHME3; Fig. 4c ), and Kif5B was also found to be required for infection of T-cell lines, Jurkat ( Fig. 4e ) and 174xCEM ( Supplementary Fig. 4a ). WB analysis confirmed Kif5 knockdown levels ( Fig. 4b,d,f and Supplementary Fig. 4b ). Importantly, kinesin-1-depleted cells exhibited no morphological changes or indications of apoptosis compared with control siRNA-treated cells ( Supplementary Fig. 2a,b ). Kif5A or Kif5B depletion in CHME3 cells also blocked infection by HIV-1-luc pseudotyped with MuLV amphotropic envelope glycoproteins ( Fig. 4g ). Furthermore, although infection by HIV-1-VSV-G was suppressed in Kif5A- or Kif5B-depleted cells, infection by VSV itself was not inhibited ( Fig. 4h ), further suggesting an envelope-independent block specific to HIV-1 that occurred at an early post-entry stage of infection. To confirm this, cells were treated with control, Kif5A or Kif5B siRNAs followed by infection with HIV-1-VSV-G carrying a β-lactamase-Vpr fusion protein, which allows monitoring of viral penetration into the cytosol [23] . Compared with control siRNA-treated samples, depletion of either Kif5A or Kif5B did not significantly affect fusion of HIV-1 into the cytoplasm of NHDFs ( Fig. 4i ), and did not correlate with the potent inhibition of early HIV-1 infection in cells depleted of either isoform ( Fig. 4a–f ). To further determine the point in the viral life cycle affected by kinesin-1, CHME3 cells were treated with control, Kif5A or Kif5B siRNAs. Cultures were then infected and levels of minus-strand strong stop (MSS) DNA, total viral DNA and 2-long terminal repeat (2-LTR) circles were determined [9] . Quantitative real-time PCR analysis of viral DNA showed that although Kif5A or Kif5B depletion did not affect MSS or total viral DNA, 2-LTR circles were potently reduced ( Fig. 4j ), suggesting a block after reverse transcription but before nuclear entry of viral DNA. This block to 2-LTR circles was also observed in CHME3 cells expressing a GFP-tagged dominant-negative form of Kif5B [24] , compared with GFP control ( Fig. 4k,l ). These findings demonstrated that kinesin-1 did not affect fusion of HIV-1 into the cytosol but was required for early post-entry stages of infection. 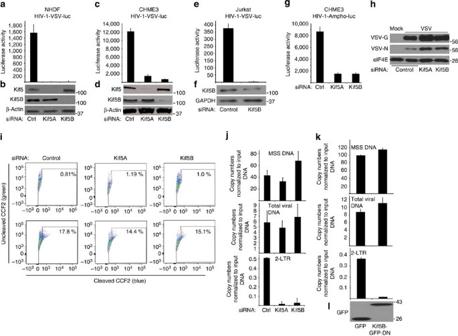Figure 4: Kinesin-1 regulates nuclear entry of HIV-1 DNA. (a–g) Kinesin-1 depletion affects early HIV-1 infection regardless of the route of viral entry. NHDF (a,b), CHME3 (c,d,g) or Jurkat (e,f) cells were transfected with control (ctrl), Kif5A or Kif5B siRNAs. Forty-eight hours post transfection, cells were infected with HIV-1-VSV-luc (a,c,e) or HIV-1-Ampho-luc (g) followed by measurements of luciferase activity in NHDF (a), CHME3 (c,g) or Jurkat (e) cells. (b,d,f). WB analysis demonstrated kinesin-1 depletion in samples froma,candeusing antibodies against kinesin-1 (Kif5A/B), Kif5B or β-actin (loading control). (h) Kinesin-1 knockdown does not inhibit VSV infection. NHDF cells treated with control, Kif5A or Kif5B siRNAs were infected 48 h post-transfection with VSV at multiplicity of infection 10. Eight hours after infection, cells were lysed and analysed by WB using anti-VSV-G or anti-VSV-N antibodies. eIF4E was used as loading control. (i) Effects of kinesin-1 depletion on fusion of HIV-1 cores into the cytosol. NHDFs were treated with control, Kif5A or Kif5B siRNAs and then either mock infected (upper panels) or infected with HIV-1-VSV-luc containing BlaM-Vpr (lower panels). FACS analysis of cells showed ~14–18% shift from green (uncleaved CCF2) to blue (cleaved CCF2) cells in control and kinesin-1-depleted cultures. (j–l) Kinesin-1 regulates nuclear entry of HIV-1 DNA. (j) CHME3 cells treated with control (Ctrl), Kif5A or Kif5B siRNAs were infected with HIV-1-VSV-puro 48 h post transfection. Low molecular Hirt DNA was isolated 24 h post infection and levels of viral MSS-DNA, total viral DNA and 2-LTRs in samples were measured by quantitative real-time PCR using specific primers to MSS, puromycin or 2-LTRs, respectively. Copy numbers were calculated and normalized to input DNA in each sample. Data are presented as mean ±s.e.m. (k,l) CHME3 cells were transfected with plasmids expressing either GFP or GFP-tagged dominant negative Kif5B (Kif5B-GFP-DN). Forty-eight hours post transfection, cells were infected (k) and levels of MSS DNA, total DN and 2-LTRs were measured as described injor (l) cells were lysed in Laemmli buffer and analysed by WB using anti-GFP antibody to detect GFP or dominant-negative GFP-Kif5 (Kif5B-GFP-DN). Molecular weight markers (in kDa) are shown to the right of WBs. Figure 4: Kinesin-1 regulates nuclear entry of HIV-1 DNA. ( a – g ) Kinesin-1 depletion affects early HIV-1 infection regardless of the route of viral entry. NHDF ( a , b ), CHME3 ( c , d , g ) or Jurkat ( e , f ) cells were transfected with control (ctrl), Kif5A or Kif5B siRNAs. Forty-eight hours post transfection, cells were infected with HIV-1-VSV-luc ( a , c , e ) or HIV-1-Ampho-luc ( g ) followed by measurements of luciferase activity in NHDF ( a ), CHME3 ( c , g ) or Jurkat ( e ) cells. ( b , d , f ). WB analysis demonstrated kinesin-1 depletion in samples from a , c and e using antibodies against kinesin-1 (Kif5A/B), Kif5B or β-actin (loading control). ( h ) Kinesin-1 knockdown does not inhibit VSV infection. NHDF cells treated with control, Kif5A or Kif5B siRNAs were infected 48 h post-transfection with VSV at multiplicity of infection 10. Eight hours after infection, cells were lysed and analysed by WB using anti-VSV-G or anti-VSV-N antibodies. eIF4E was used as loading control. ( i ) Effects of kinesin-1 depletion on fusion of HIV-1 cores into the cytosol. NHDFs were treated with control, Kif5A or Kif5B siRNAs and then either mock infected (upper panels) or infected with HIV-1-VSV-luc containing BlaM-Vpr (lower panels). FACS analysis of cells showed ~14–18% shift from green (uncleaved CCF2) to blue (cleaved CCF2) cells in control and kinesin-1-depleted cultures. ( j – l ) Kinesin-1 regulates nuclear entry of HIV-1 DNA. ( j ) CHME3 cells treated with control (Ctrl), Kif5A or Kif5B siRNAs were infected with HIV-1-VSV-puro 48 h post transfection. Low molecular Hirt DNA was isolated 24 h post infection and levels of viral MSS-DNA, total viral DNA and 2-LTRs in samples were measured by quantitative real-time PCR using specific primers to MSS, puromycin or 2-LTRs, respectively. Copy numbers were calculated and normalized to input DNA in each sample. Data are presented as mean ±s.e.m. ( k , l ) CHME3 cells were transfected with plasmids expressing either GFP or GFP-tagged dominant negative Kif5B (Kif5B-GFP-DN). Forty-eight hours post transfection, cells were infected ( k ) and levels of MSS DNA, total DN and 2-LTRs were measured as described in j or ( l ) cells were lysed in Laemmli buffer and analysed by WB using anti-GFP antibody to detect GFP or dominant-negative GFP-Kif5 (Kif5B-GFP-DN). Molecular weight markers (in kDa) are shown to the right of WBs. Full size image Dynein and kinesin-1 are necessary for early HIV-1 infection It has been shown previously that in some cellular contexts the inhibition of kinesin-1 activity can result in the accumulation of dynein at the trans-golgi network (TGN) [25] , [26] . This might also explain the block to early HIV-1 infection. To test this, the levels and distribution of dynein in cells treated with control, Kif5A or Kif5B siRNAs were examined. WB analysis revealed that Kif5A or Kif5B depletion did not affect the levels of dynein or β-actin compared with control samples ( Fig. 5a ). Furthermore, immunofluorescence (IF) analysis of fixed cells stained using antibodies against Kif5, dynein intermediate chain (IC74) and the TGN marker, TGN46, revealed no notable differences in the distribution of dynein between cells treated with control or kinesin-1-specific siRNAs, nor were increases in dynein accumulation at the TGN detected ( Fig. 5b ). These findings demonstrated that the block to HIV-1 infection in kinesin-1-depleted cells was not due to defects in dynein levels or localization. 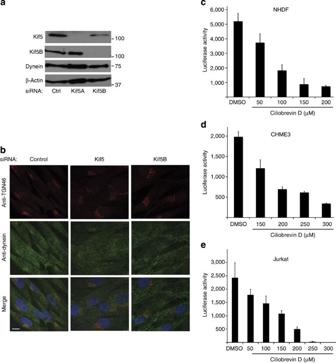Figure 5: Kinesin-1 depletion does not affect dynein, an inward motor required for HIV-1 infection. (a,b) Effects of kinesin-1 depletion on dynein levels and distribution. NHDF cells were treated with control siRNA (Ctrl) or siRNAs targeting Kif5A or Kif5B. Forty-eight hours post transfection, cells were either lysed and analysed by WB (a) or fixed and stained (b) using antibodies to kinesin-1 (Kif5A/B), Kif5B, dynein, trans-golgi network marker (TNG46) or β-actin. Molecular weight markers (in kDa) are shown to the right of WBs. Scale bars represent 10 μm. (c–e) Dynein is required for early HIV-1 infection. NHDF (c), CHME3 (d) or Jurkat (e) cells were treated with the indicated concentrations of the dynein inhibitor Ciliobrevin D for 30 min followed by HIV-1-VSV-luc infection in the presence of inhibitor. Luciferase activity was measured 48 h post infection to determine levels of infection. Error bars represent standard deviation from three independent experiments. Figure 5: Kinesin-1 depletion does not affect dynein, an inward motor required for HIV-1 infection. ( a , b ) Effects of kinesin-1 depletion on dynein levels and distribution. NHDF cells were treated with control siRNA (Ctrl) or siRNAs targeting Kif5A or Kif5B. Forty-eight hours post transfection, cells were either lysed and analysed by WB ( a ) or fixed and stained ( b ) using antibodies to kinesin-1 (Kif5A/B), Kif5B, dynein, trans-golgi network marker (TNG46) or β-actin. Molecular weight markers (in kDa) are shown to the right of WBs. Scale bars represent 10 μm. ( c – e ) Dynein is required for early HIV-1 infection. NHDF ( c ), CHME3 ( d ) or Jurkat ( e ) cells were treated with the indicated concentrations of the dynein inhibitor Ciliobrevin D for 30 min followed by HIV-1-VSV-luc infection in the presence of inhibitor. Luciferase activity was measured 48 h post infection to determine levels of infection. Error bars represent standard deviation from three independent experiments. Full size image Although our findings demonstrated that kinesin-1 was important for early HIV-1 infection, previous reports have shown dynein-dependent trafficking of HIV-1 towards the nucleus [4] , [5] . To test whether this was also the case in our cell systems, and whether both inward and outward motors were important for early HIV-1 infection, human microglia (CHME3), primary human cells (NHDFs) and T cells (Jurkat) were treated with various concentrations of the dynein inhibitor, ciliobrevin D [27] , followed by infection with HIV-1-VSV-luc. When luciferase reporter gene expression was measured, a dose-dependent inhibition of infection was detected in all three cell types treated with ciliobrevin D compared with dimethylsulphoxide-treated controls ( Fig. 5c–e ). This demonstrated that in the inward motor, dynein was required for early HIV-1 infection of microglia, T cells and primary human fibroblasts, similar to the previous reports [4] , [5] . Overall, our combined findings demonstrated that both inward and outward motors are necessary for early HIV-1 infection. Kinesin-1 functions in FEZ-1-mediated HIV-1 trafficking To determine whether kinesin-1 affected the movement of HIV-1 particles towards the nucleus, NHDFs were treated with control, Kif5A or Kif5B siRNAs and then infected with HIV-1-GFP-Vpr. Live imaging revealed that depletion of either isoform of kinesin-1 potently inhibited the movement of virus towards the nucleus compared with control siRNA-treated samples ( Fig. 6a and Supplementary Movies 5–7 ). These effects were further confirmed by quantification of the total number of particles within 2 μm of the nucleus over time ( Fig. 6b ), which showed that the vast majority of viral particles failed to traffic towards the nucleus in kinesin-1-depleted cells. Furthermore, in kinesin-1-depleted cells virus particles exhibited movements characteristic of either free diffusion in the cytosol or actin-mediated movement. These observations were in line with results from fusion and viral DNA synthesis assays ( Fig. 4i–l ), and suggested that in kinesin-1-depleted cells virus particles entered the cytosol but were only capable of short-ranged movements largely at the cell periphery. Furthermore, the requirement for kinesin-1 to facilitate trafficking of HIV-1 to the nucleus suggested that FEZ1’s function as a kinesin-1 adaptor protein might underlie FEZ1’s role in early infection. To test this, we examined the effects on HIV-1 infection of exogenous expression of FEZ1 or a recently described FEZ1 mutant, FEZ1-S58A [28] . This mutant, where serine 58 is replaced with alanine, fails to bind kinesin-1 in Caenorhabditis elegans [28] . To confirm this for their human counterparts, GFP control or a GFP-tagged form of human kinesin-1 heavy chain tail [24] (containing the FEZ1-binding domain [28] ) was expressed in cells along with FEZ1-Flag or FEZ1-S58A-Flag. GFP was then recovered from cell extracts using sepharose-conjugated GFP-binding peptide [29] . Binding assays showed that FEZ1-Flag did not bind GFP but specifically bound Kif5B, whereas the S58A mutation abolished this binding ( Fig. 7a ). Stable pools of NHDFs expressing Flag control, FEZ1-Flag or FEZ1-S58A-Flag were then generated, and equal expression of exogenous forms of FEZ1 was confirmed by WB analysis ( Fig. 7b ). Infection of these pools with HIV-1-VSV-luc reporter revealed that exogenous expression of FEZ1-Flag enhanced HIV-1 infection, whereas FEZ1-S58A-Flag did not increase infection above that of Flag control cells ( Fig. 7c ). The same results were observed when pools were infected with HIV-1-luc reporter virus pseudotyped with MuLV amphotropic envelope ( Fig. 7d ), demonstrating that these effects were again independent of the route of viral entry. Importantly, both FEZ1-Flag and FEZ1-S58A-Flag bound in vitro assembled HIV-1 CA–NC equally ( Fig. 7e ). These interactions were also confirmed by co-transfection of 293A cells with either FEZ1-Flag or FEZ1-S58A-Flag along with a HIV-1 Gag-expressing vector. Similar to CA–NC assays both forms of FEZ1 were found to Co-IP with HIV-1 Gag ( Fig. 7f ). Overall, these findings demonstrated that kinesin-1 was required for viral movement to the nucleus and that FEZ1’s ability to bind kinesin-1 was required for this HIV-1-associated adaptor protein to regulate early stages of HIV-1 infection. 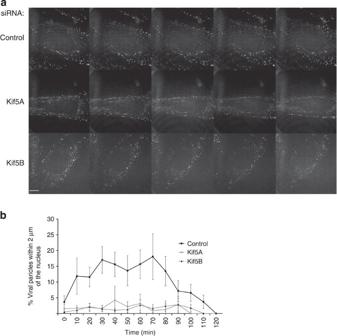Figure 6: Depletion of kinesin-1 inhibits trafficking of HIV-1 particles to the nucleus. NHDFs were treated with control siRNA or siRNAs targeting either of two different isoforms of kinesin-1 heavy chain (Kif5A or Kif5B). Forty-eight hours post transfection cells were infected with HIV-1-VSV-GFP-Vpr followed by live imaging of particle movement. (a) Still images from movies (Supplementary Movies 5–7) at the indicated time points are shown. Scale bars represent 10 μm. (b) Quantification of the percentage of virions within 2 μm of the nucleus in infected cells at the indicated time points.n≥15 cells and an average of 53–91 viral particles per cell. Results are representative of three or more independent experiments, and error bars represent standard deviation. Figure 6: Depletion of kinesin-1 inhibits trafficking of HIV-1 particles to the nucleus. NHDFs were treated with control siRNA or siRNAs targeting either of two different isoforms of kinesin-1 heavy chain (Kif5A or Kif5B). Forty-eight hours post transfection cells were infected with HIV-1-VSV-GFP-Vpr followed by live imaging of particle movement. ( a ) Still images from movies ( Supplementary Movies 5–7 ) at the indicated time points are shown. Scale bars represent 10 μm. ( b ) Quantification of the percentage of virions within 2 μm of the nucleus in infected cells at the indicated time points. n ≥15 cells and an average of 53–91 viral particles per cell. Results are representative of three or more independent experiments, and error bars represent standard deviation. 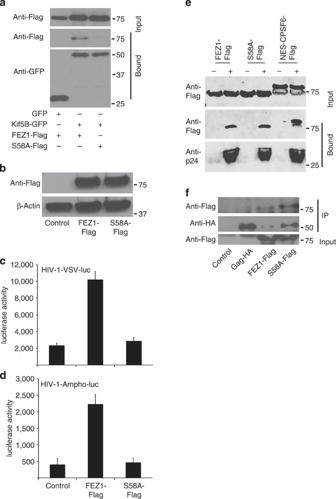Figure 7: Binding to kinesin-1 is required for FEZ1 to promote early HIV-1 infection. (a) 293A cells were transfected with vectors expressing a control GFP or GFP-Kif5B tail along with either FEZ1-Flag or FEZ1-S58A-Flag (S58A-Flag) constructs. Soluble cell extracts were prepared 48 h post transfection, precleared and GFP proteins were recovered by incubating samples with GFP-binding protein (GBP) covalently coupled to Sepharose. Input and bound proteins were then analysed by WB using anti-Flag and anti-GFP antibodies. (b) Pools of NHDF cells stably expressing Flag control (Control), full-length C-terminally flag-tagged FEZ1 (FEZ1-Flag) or a C-terminally flag-tagged FEZ1 mutant unable to bind kinesin-1 (S58A-Flag) were lysed and analysed by WB using antibodies against Flag or β-actin (loading control). (c,d) NHDF pools described inbwere infected with HIV-1-VSV-luc (c) or HIV-1-Ampho-luc (d) followed by measurements of luciferase activity 48 h post infection to determine levels of infection. Results are representative of three or more independent experiments, and error bars represent standard deviation. (e) Binding of FEZ1 or FEZ1-S58A toin vitroassembled HIV-1 CA–NC complexes. 293T cells were transfected with FEZ1-Flag, FEZ1-S58A-Flag (S58a-Flag) or NES-CPSF6-Flag constructs as described in the legend forFig. 2. Cells were lysed 36 h post transfection and the lysates were incubated at room temperature for 1 h within vitroassembled HIV-1 CA–NC complexes. The lysates were then analysed by WB either before (input) or after sedimentation through a 70% sucrose cushion (bound) using anti-Flag and anti-p24 antibodies. (f) Binding of FEZ1-S58A to HIV-1 Gag by Co-IP. 293A cells were co-transfected with a HA-tagged HIV-1 Gag-expressing vector alone or together with FEZ1-Flag or FEZ1-S58A-Flag (S58A-Flag). Cells were lysed 48 h post transfection, and proteins were co-IP using anti-HA antibodies. Input and bound samples were then analysed by WB either before (input) or after immunoprecipitation (IP) using anti-Flag and anti-HA antibodies. Molecular weight markers (in kDa) are shown to the right of WBs. Full size image Figure 7: Binding to kinesin-1 is required for FEZ1 to promote early HIV-1 infection. ( a ) 293A cells were transfected with vectors expressing a control GFP or GFP-Kif5B tail along with either FEZ1-Flag or FEZ1-S58A-Flag (S58A-Flag) constructs. Soluble cell extracts were prepared 48 h post transfection, precleared and GFP proteins were recovered by incubating samples with GFP-binding protein (GBP) covalently coupled to Sepharose. Input and bound proteins were then analysed by WB using anti-Flag and anti-GFP antibodies. ( b ) Pools of NHDF cells stably expressing Flag control (Control), full-length C-terminally flag-tagged FEZ1 (FEZ1-Flag) or a C-terminally flag-tagged FEZ1 mutant unable to bind kinesin-1 (S58A-Flag) were lysed and analysed by WB using antibodies against Flag or β-actin (loading control). ( c , d ) NHDF pools described in b were infected with HIV-1-VSV-luc ( c ) or HIV-1-Ampho-luc ( d ) followed by measurements of luciferase activity 48 h post infection to determine levels of infection. Results are representative of three or more independent experiments, and error bars represent standard deviation. ( e ) Binding of FEZ1 or FEZ1-S58A to in vitro assembled HIV-1 CA–NC complexes. 293T cells were transfected with FEZ1-Flag, FEZ1-S58A-Flag (S58a-Flag) or NES-CPSF6-Flag constructs as described in the legend for Fig. 2 . Cells were lysed 36 h post transfection and the lysates were incubated at room temperature for 1 h with in vitro assembled HIV-1 CA–NC complexes. The lysates were then analysed by WB either before (input) or after sedimentation through a 70% sucrose cushion (bound) using anti-Flag and anti-p24 antibodies. ( f ) Binding of FEZ1-S58A to HIV-1 Gag by Co-IP. 293A cells were co-transfected with a HA-tagged HIV-1 Gag-expressing vector alone or together with FEZ1-Flag or FEZ1-S58A-Flag (S58A-Flag). Cells were lysed 48 h post transfection, and proteins were co-IP using anti-HA antibodies. Input and bound samples were then analysed by WB either before (input) or after immunoprecipitation (IP) using anti-Flag and anti-HA antibodies. Molecular weight markers (in kDa) are shown to the right of WBs. Full size image Many viruses, including retroviruses such as HIV-1, hijack their hosts’ MT transport system at various stages of their life cycle in order to successfully replicate and spread. Despite this, the viral and cellular factors, and the mechanisms involved in MT-based trafficking of HIV-1 towards the nucleus remain poorly understood. Here we show that the kinesin-1 adaptor protein FEZ1 interacts with in vitro assembled HIV-1 capsid-nucleocapsid complexes and regulates HIV-1 movement towards the nucleus. Furthermore, we show that both kinesin-1 and dynein are required for viral trafficking to the nucleus. Our findings suggest a model whereby motors of opposing directionality regulate each other’s activity and that incoming HIV-1 binds and usurps the kinesin-1 adaptor protein, FEZ1 to regulate this process to accomplish net forward movement towards the nucleus. Previously, we showed that FEZ1 was naturally expressed at high levels in neurons compared with other brain cell types and that FEZ1 was a contributing factor to neuronal resistance to HIV-1 infection [9] . FEZ1 has also been shown to negatively affect infection of a transformed glia cell line by the human polyomavirus JC virus, although the underlying mechanism remains unknown [30] . Here, we show that levels of FEZ1 are much lower in human microglia, monocytes, T cells and primary normal human fibroblasts than in neurons, and that endogenous FEZ1 in non-neuronal cells plays a positive role in infection. Combined with the mechanistic insights into FEZ1’s function during infection provided here, and discussed below, these findings radically change our view of FEZ1 from that of an antiviral factor highly expressed in neurons to a positive host cofactor exploited by the virus to facilitate infection. There are several reasons that could explain our original observations in neurons. For example, FEZ1 may be differently modified or associated with a very different set of accessory proteins in neurons, altering its behaviour or HIV-1’s ability to exploit its activity in these cells. Alternatively, excessively high levels of FEZ1 expression may simply saturate incoming viral particles or throw off stoichiometries with other co-factors that may be critical to FEZ1’s function in HIV-1 infection. On this point, we have previously shown that overexpression of FEZ1 in CHME3 microglia suppresses HIV-1 infection [9] , yet here we show that depletion of endogenous FEZ1 in the same cells also inhibits infection. In working with these cells, we have found that modest overexpression of FEZ1 in CHME3 cells can modestly stimulate infection, but that higher levels of overexpression quickly become a negative factor for infection. This suggests that in CHME3 cells endogenous FEZ1 levels are close to a threshold of becoming negative, similar to neurons. A very similar situation exists for the P-body component Mov10 wherein either depletion or overexpression can negatively impact HIV-1 infection [31] . In line with this concept, we also show here that exogenous FEZ1 promotes HIV-1 infection in NHDFs but reaches a saturating point where further increases in expression begin to reduce infection. All of our core findings using NHDFs validate in a variety of natural target cell types, including microglia, macrophages and T cells. To this end, we have found that primary NHDFs offer a robust FEZ1-responsive cell system to study these events in a normal cell background, rather than using transformed cell lines that contain many aberrant regulatory pathways. Overall, our findings clearly establish that FEZ1 is a positive factor for infection in normal human cells, macrophages and in microglia, the key target cell for HIV-1 infection in the central nervous system associated with the neurodegeneration seen in patients with HIV-associated dementia [32] . Our findings not only redefine the view that FEZ1 acts as an antiviral factor for HIV-1 but also uncover the mechanistic basis for how FEZ1 regulates HIV-1 infection. Our previous studies showed that FEZ1 did not affect viral entry into the cell but blocked the accumulation of retroviral DNA in the nucleus [8] , [9] . FEZ1 overexpression can affect nuclear architecture [33] , [34] , [35] , [36] , [37] , [38] , [39] , suggesting that FEZ1 might influence HIV-1 nuclear entry. Findings here, however, show that FEZ1 depletion also blocks infection by viral mutants that bypass known HIV-1 nuclear entry pathways [18] , demonstrating that FEZ1 does not influence HIV-1 nuclear entry pathways specifically. Although broader effects on multiple nuclear entry pathways remain a possibility, our results show that the primary effect of FEZ1 is on the trafficking of HIV-1 particles to the nucleus. FEZ1 acts as a cargo adaptor protein, with its C-terminus mediating interactions with other proteins, whereas its N-terminus is important for its dimerization [40] , [41] . Dimerization is thought to be important for FEZ1’s biological function, possibly allowing simultaneous binding to cytoskeletal elements and cargos [42] . FEZ1 also binds and regulates the activity of the MT motor protein kinesin-1 and this is thought to play a role in the transport of vesicles and organelles along MTs in neurons [20] , [28] , [43] , [44] , [45] , [46] , [47] . In line with this motor adaptor function of FEZ1, live imaging revealed that FEZ1 is required for HIV-1 particles to traffic to the nucleus. In the absence of FEZ1, virus particles exhibited bi-directional movement suggestive of alternating activity of inward and outward motors, but which ultimately resulted in no net movement to the nucleus. Notably, previous studies have shown that HIV-1 exhibits bi-directional motility [4] , [5] , and we observe the same behaviour in normal human fibroblasts and microglia. Furthermore, inhibition of dynein by anti-dynein antibody microinjection or expression of a dominant negative inhibitor of dynactin causes incoming viral particles to accumulate at the cell periphery rather than diffuse through the cytoplasm [4] , [5] . These observations have lead to the suggestion that HIV-1 particles can associate with both dynein and kinesin [48] . Indeed, a number of viruses that traffic to the nucleus, including adenovirus [49] and herpes simplex type 1 (refs 50 , 51 , 52 , 53 ), also bind motors of opposite polarity and exhibit bi-directional motility. Several models have been proposed for how viruses bound by opposing motors accomplish net directed movement to the nucleus [48] , [54] . For some it has been proposed that they bind motors of opposite polarity sequentially and undergo a stochastic ‘tug of war’, with virus particles ultimately reaching the nucleus randomly, or that motor binding is cell-type dependent. Viruses can also influence motor activity. Adenovirus, for example, stimulates both PKA and p38 signalling to activate dynein-mediated minus end-directed motility [49] , [55] , [56] . For others it has been suggested that localized control of motor binding or motor activity might regulate directed movement, although this has never been directly demonstrated. Even if precise regulatory mechanisms remain unclear, dynein has been shown to be required for inward movement of many viruses towards the nucleus. However, the potential role or effect of kinesin binding by incoming viral particles remains poorly understood. In the case of adenovirus, kinesin-1 has been shown to promote capsid uncoating and nuclear pore complex disruption to promote viral DNA entry into the nucleus [57] . Using a specific dynein inhibitor, we confirmed previous reports of the requirement for dynein for early HIV-1 infection in primary NHDFs, microglia and T cells. Perhaps more surprisingly, and distinct from adenovirus, we find that kinesin-1 is also required for early HIV-1 infection in all three cell types. In the absence of kinesin-1, viral particles enter the cell but remain at the cell periphery exhibiting motility reminiscent of free diffusion or actin-based motion. Notably, while this paper was under review a report showed that a siRNA targeting Kif5B resulted in delayed uncoating [58] , although no mechanism was provided beyond this observation. Our finding that HIV-1 requires kinesin-1 to move to the nucleus offers a mechanistic explanation for this observation, as uncoating is thought to occur either during trafficking to or upon arrival at the nucleus [4] , [5] , [6] . Our findings further establish that incoming HIV-1 particles require both dynein and kinesin for MT-dependent trafficking from the cell surface to the nucleus. The regulatory interactions between opposing motors on the same cargo are complex and while opposing motors can compete, they can also regulate each other’s activity. Indeed, knockdown of a motor of one polarity (minus- or plus-end directed) has been shown to result in a complete block in the bi-directional motility of some cargos [59] . Our observation that depletion of kinesin-1 blocks MT-dependent movement of HIV-1 particles is in line with these observations. In addition, several adaptor molecules have been shown to bind to motors of opposite polarity to regulate their activity [26] . Again, in line with these observations, we find that HIV-1 particles bind to the kinesin-1 adaptor protein, FEZ1, and establish that kinesin-1 binding is necessary for FEZ1 to promote infection. It is intriguing to think of this as an example of localized viral manipulation of motor function through binding to a host adaptor protein. Although two reports have suggested interactions with dynein components for other retroviruses [60] , [61] , no such interactions have been reported for HIV-1 to date. In terms of broader interactions with motors, kinesins have been shown to function in the late stages of infection by several retroviruses [62] , and specifically Gag and Matrix proteins of HIV-1 have been shown to interact with the kinesin, Kif4, which mediates release of virus-like particles that mimic late stages of infection [63] , [64] . However, whether this involves Kif4 motor activity remains unclear, as Kif4 also functions to stabilize MT networks as the virus enters the cell [65] . Indeed, another kinesin, Kif3A, has been shown to also function in HIV-1 release [66] , [67] . Overall, how HIV-1 interacts with the MT motor machinery of the cell has remained somewhat elusive. Our findings suggest that HIV-1 capsids bind FEZ1 to enable the virus to regulate its motility after entering the cell, but this may also provide a means for viral particles to connect indirectly to motor proteins or motor complexes. Such indirect interactions may also explain why it has proven challenging to detect motors on HIV-1 particles. Overall, we show that both inward and outward motors are important for HIV-1 trafficking to the nucleus and uncover how viral particles bind and usurp the activity of a host kinesin-adaptor, FEZ1, to regulate bi-directional motility to accomplish net transport to the nucleus. Cells and viruses NHDFs were purchased from Lonza. 293T, 293A and CHME3 cells were described previously [8] . H9 and 174xCEM were provided by AIDS Reagent Repository (number 87 and 272, respectively). The following T-cell lines and monocytic lines were kindly provided by Thomas Hope (Jurkat, U937 and Thp-1), Chyung-Ru Wang (Molt-4, K562) and Hyewon Phee (HUT78). Thp-1 cells were differentiated to macrophages by the addition of phorbol myristate acetate (PMA) (30 ng ml −1 ) to cultures overnight. To generate HIV-1 carrying a luciferase reporter, pNL4-3.Luc.R − .E − plasmid (AIDS Reagent Repository number 3418) [68] was transfected into 293T cells together with constructs expressing VSV-G (PMDG) or MuLV amphotropic (pHit456) envelope glycoprotein [65] . Forty-eight hours post transfection, culture supernatants were harvested as described [65] . Vpr-labelled viruses were generated by co-transfection with GFP-Vpr plasmid [4] , [65] . GFP-Vpr/S15-Tomato-labelled virus was generated using 5.7 mg of pNL4-3.Luc.R − .E − , 2.9 mg of VSV-g, 1.4 mg of GFP-Vpr and 0.44 mg of S15-Tomato as described [21] . HIV-1 WT or capsid mutants were generated using PMDG and the luciferase-expressing vector pHR’-CMV-luciferase [69] together with retroviral vectors expressing either Gag-Pol containing WT capsid (p8.91) or mutant capsid (N74D or P90A) [19] . Total numbers of HIV-1 WT or capsid mutants in preparations were estimated by serial dilution of virus and analysis of p24 levels by ELISA. Infections and fusion assays NHDFs or CHME3 cells seeded in 12-well plates were infected with different dilutions of HIV-1-VSV-luc or HIV-1-Ampho-luc as described [65] . Cells were lysed 48–72 h post infection (h.p.i.) and assayed for luciferase activity. Virion-based fusion assays using HIV-1-VSV-luc containing the BlaM-Vpr fusion protein (AIDS Reagent Repository number 3418) [68] were described previously [23] , [65] . Infections with GFP-Vpr- or GFP-Vpr/S15-Tomato-labelled HIV-1 were performed in CO 2 -independent medium (Life Technologies, 18045-088) supplemented with 10% FBS, 1 mM sodium pyruvate and 2 mM glutamine for 2 h at 13 °C via spinoculation [21] . For experiments with Bafilomycin A1 (Sigma), the drug was prepared in dimethylsulphoxide and diluted to a final concentration of 20 nM in DMEM. Vesicular Stomatitis Virus (Indiana strain) was grown on BSC40 cells and viral titres were determined on both BSC40 cells and NHDFs. Western blotting and IF Antibodies were obtained from the following sources: anti-FEZ1 (Sigma, HPA038490); anti-Flag (Sigma, F7425); anti-β actin (Sigma, clone AC-15/A1978); anti-HIV-1 p24 (Abcam, ab9071); anti-Kinesin (Abcam, ab25715); anti-Kif5B (Abcam, ab15705); anti-dynein intermediate chain (Millipore, clone 74.1, MAB1618) and anti-TNG46 (AbD Serotec, AHP500), anti-eIF4E (BD Biosciences, 610269), anti-GFP (Abcam, ab13970), anti-GAPDH (Santa Cruz, sc-25778), anti-HA (Sigma, H6098), anti-VSV-G (Abcam, ab50549), anti-VSV-N (KeraFAST, EB0009) and anti-PARP (Cell Signaling, 9542). For WB analysis, all primary antibodies were used at 1:1,000 dilution (except anti-β actin; 1:2,500) and detected using the appropriate HRP-conjugated secondary antibodies. Uncropped scans of the most important blots are shown in Supplementary Figs 6–9 . Where relative protein levels were compared in experimental setups, bands from scanned film were demarcated on inverted images and the sum of pixel grey values was measured using ImageJ software. Numbers were normalized to corresponding loading control proteins. For IF analysis, cells grown on glass coverslips were fixed with 3.7% paraformaldehyde, blocked and permeabilized as described [65] . Samples were incubated with primary antibody overnight at 4 °C, washed and incubated with the appropriate Alexa Fluor-conjugated secondary for 1 h at room temperature. Dilutions for primary antibodies were: 1:150 anti-TGN46, 1:200 anti-kinesin and 1:500 anti-dynein intermediate chain. Nuclei were stained with Hoechst 33342. Cells infected with GFP-Vpr/S15-Tomato-labelled virions were stained with Hoechst 33342 in PBS/0.1% saponin and mounted with FluorSave reagent (Calbiochem). Images were acquired using a Zeiss LSM 710 confocal laser scanning microscope or a motorized spinning-disc confocal microscope (Zeiss Axio Observer Z1 or Leica DMI 6000B) with Yokogawa CSU-X1 A1 confocal head. Live imaging and analysis Live-cell video microscopy was performed using a motorized spinning-disc confocal microscope (described above) and environmental chamber (3i Intelligent Imaging Innovations or InVivo Scientific). Cells were plated on collagen-coated glass 35-mm culture dishes (MatTek, P35G-1.5-14C). Before imaging, cells were washed once and supplemented with fresh medium containing the oxygen scavenger Oxyrase (Oxyrase Company) to reduce photodamage and photobleaching and imaged in an environmental chamber at 37 °C. Images were acquired with a Photometrics Evolve 512 EMCCD camera driven by SlideBook Software (3i Intelligent Imaging Innovations) or with a Hamamatsu ImagEM X2 EMCCD camera run by MetaMorph imaging software (Molecular Devices). Particle tracking was analysed with Diatrack version 3.01 software (Semasopht) using vector analysis. Images were captured every 0.5 s for a period of 2.5 min. Vectors were defined as displacement between two consecutive frames. They were split into trajectories to or from nucleus. Trajectories of each direction were summed and divided by the mean number of particles in the analysed areas of the image; this calculation gives the distance travelled per particle. The threshold speed was 0.2 μm s −1 in order to exclude actin-dependent movements. All particles with lifetime less than 1.5 s were excluded from the calculations. At least two independent experiments were analysed for each condition, and each experiment consisted of five cells with between 7 and 30 particles per cell. The number of GFP-positive virions was assessed and each virion was individually inspected for punctate Tomato fluorescent signal. Between 23 and 30 images were analysed for each data point provided. During analysis, channel intensity was increased above the level of the included figures to detect low-level fluorescence. RNA interference and dominant negative expression For transient knockdown, CHME3 or NHDF cells were transfected with siRNA duplexes using oligofectamine RNAiMAX transfection reagent (Invitrogen) as described [9] . siRNAs used were: ID# 45012 (FEZ1-B), ID# 45101 (FEZ1-C), ID# s7837 (Kif5A), siRNA ID# s731 (Kif5B), ID# AM4635 (control non-targeting siRNA) or a control siRNA duplex targeting GFP from Ambion. Cells were transfected on two consecutive days with 300 pmol of siRNA duplex or 60 pmol of siRNA Select duplexes, then infected with HIV-1-VSV-luc or HIV-1-Ampho-luc. Cells were then lysed and luciferase activity was measured as described above. Jurkat and 174xCEM T cells were seeded in a 12-well plate at 3 × 10 5 cells per well or in a 6-well plate at 2 × 10 5 cells per well, respectively. Cells were then transfected with 60 pmol of siRNA Select duplexes using RNAiMAX. Forty-eight hours post transfection, Jurkat cells were infected with HIV-1-VSV-luc at 1:500 dilution of the neat virus, whereas 174xCEM cells were seeded in a 12-well plate at 5 × 10 4 cells per well before infection with HIV-1-VSV-luc at 1:500 dilution. Two days after infection cells were lysed and assayed for luciferase activity. For macrophage studies, 2 × 10 5 Thp-1 cells were plated per well of 12-well plate and differentiated to macrophages with PMA as described above. Twenty-four hours later, cultures were washed twice and differentiated cells were maintained in complete media with no antibiotics for a further 24 h. Cultures were then transfected with 300 pmol siRNA and 48 h later infected with HIV1-VSV-luc. Luciferase activity was measured 40 h.p.i. For expression of dominant negative GFP-Kif5B or GFP control, CHME3 cells were seeded at 3.5 × 10 5 cells in a 60-mm dish. The following day the media were replaced with DMEM without antibiotics or FBS 3 h before transfection. Transfection was performed using 2 μg DNA and 4 μl lipofectamine 2000 (Life Technologies) as per manufacturer’s instructions. Cells were then infected and processed as described in the text. In vitro capsid-binding assay The HIV-1 CA–NC expression, purification and assembly were performed as previously described [14] . HIV-1 CA–NC particles were assembled in vitro by diluting the CA–NC protein to a concentration of 10 mg ml −1 in 50 mM Tris-HCl (pH 8.0), 0.5 M NaCl and 2 mg ml −1 DNA oligo-(TG)50 as described [70] . For binding of FEZ1 variants to in vitro assembled HIV-1 CA–NC complexes, human 293T cells were transfected with a previously described mammalian expression vector encoding C’ terminally Flag-tagged FEZ1 (ref. 9 ), C’ terminally Flag-tagged S58A (a mutant version of FEZ1), C’ terminally Flag-tagged NES-CPSF6 (ref. 15 ) or C’ terminally Flag-tagged SAMHD1 (ref. 17 ). Cell lysates were made and incubated with in vitro assembled CA–NC (input) followed by ultra centrifugation through a 70% sucrose cushion and resuspension of the pellet in SDS–PAGE loading buffer (Bound), as described previously [15] . WB analysis was used to determine the levels of FEZ1, NES-CPSF6 and SAMHD1 in lysates and bound to in vitro assembled capsids using anti-Flag antibodies. Pelleting of capsids in samples was confirmed by WB analysis of HIV-1 CA–NC protein using anit-p24 antibody. Expression constructs and stable pools Generation of a MuLV-based retroviral vector pQCXIN (Clontech) encoding full-length C’-terminally flag-tagged human FEZ1 (FEZ1-Flag) or the control Flag (Flag) were described previously [9] . FEZ1-S58A-Flag (serine to alanine substitution at site 58) was generated using FEZ1-Flag [9] as template and a Quickchange site-directed mutagenesis kit (Agilent Technologies). Primers used were: Sense 5′- GAAATAATCAGCTTCAAGGCCATGGAGGACCTCGTAA -3′ and Antisense 5′- TTACGAGGTCCTCCATGGCCTTGAAGCTGATTATTTC -3′. The serine to alanine substitution was confirmed by sequencing. These retroviral vectors were then used to generate VSV-G pseudotyped MuLV-expressing Flag, FEZ1-Flag or FEZ1-S58A-Flag by co-transfection of 293T cells as previously described [9] . NHDF cells were then infected with these viruses and pools of stably expressing Flag, FEZ1-Flag or FEZ1-S58A-Flag were generated by drug selection. Quantitative real-time PCR measurement of viral DNA To quantify viral DNA, CHME3 cells were infected at high multiplicity of infection with HIV-1-VSV-puro as described [9] . Hirt DNA was isolated at 24 h post infection and the amount of HIV-1 MSS-DNA, total viral DNA and 2-LTR circles were measured using primers specific to MSS, puromycin and 2-LTRs, respectively. The number of target copies were calculated using standard curves as described previously [9] . Co-immunoprecipitation and kinesin-1-binding assays For Co-IP analysis of Gag and FEZ1 interactions, 293A cells were seeded at 3 × 10 5 cells in a 60-mm dish. The following day cells were co-transfected with equimolar amounts of a HIV-1 Gag-HA-expressing vector [65] alone or together with FEZ1-Flag or FEZ1-S58A-Flag using 10 μl Turbofect (Thermo Scientific) as per manufacturer’s instructions. Cells were lysed 48 h post-transfection in NP40 lysis buffer containing protease inhibitors for 40 min at 4 °C (ref. 65 ) and pre-cleared. Input samples were taken and remaining extracts were immunoprecipitated using anti-HA antibody for 1 h at 4 °C. Immune complexes were recovered by incubating samples with protein A Sepharose for 1 h at 4 °C. Beads were then washed extensively in NP-40 lysis buffer and boiled in Laemmli buffer [65] . For kinesin-1-binding assays, 293A cells were seeded at 1 × 10 6 cells in a 100-mm dish in DMEM without antibiotics. The next day, cells were co-transfected with equimolar amounts of FEZ1-Flag- or FEZ1-S58A-Flag-expressing vectors along with either a GFP-expressing control vector or a construct encoding a GFP-tagged Kif5B-tail domain [24] using 28 μl Turbofect (Thermo Scientific) as per manufacturer’s instructions. Forty-eight hours post transfection cells were lysed in 1 ml cold NP-40 lysis buffer supplemented with Complete mini protease inhibitor tablets (Roche) [65] rocking for 40 min at 4 °C. Extracts were centrifuged at 10,000 g for 10 min at 4 °C and pre-cleared with Sepharose beads. Input samples were taken and the remaining pre-cleared extract was incubated with GFP-binding protein covalently coupled to Sepharose for 4 h at 4 °C (ref. 29 ). Beads were extensively washed in NP40 lysis buffer and bound proteins were eluted with SDS sample buffer and analysed by WB using anti-GFP and anti-Flag antibodies. How to cite this article: Malikov, V. et al . HIV-1 capsids bind and exploit the kinesin-1 adaptor FEZ1 for inward movement to the nucleus. Nat. Commun. 6:6660 doi: 10.1038/ncomms7660 (2015).